Graphene-modified nanostructured vanadium pentoxide hybrids with extraordinary electrochemical performance for Li-ion batteries The long-standing issues of low intrinsic electronic conductivity, slow lithium-ion diffusion and irreversible phase transitions on deep discharge prevent the high specific capacity/energy (443 mAh g −1 and 1,550 Wh kg −1 ) vanadium pentoxide from being used as the cathode material in practical battery applications. Here we develop a method to incorporate graphene sheets into vanadium pentoxide nanoribbons via the sol–gel process. The resulting graphene-modified nanostructured vanadium pentoxide hybrids contain only 2 wt. % graphene, yet exhibits extraordinary electrochemical performance: a specific capacity of 438 mAh g −1 , approaching the theoretical value (443 mAh g −1 ), a long cyclability and significantly enhanced rate capability. Such performance is the result of the combined effects of the graphene on structural stability, electronic conduction, vanadium redox reaction and lithium-ion diffusion supported by various experimental studies. This method provides a new avenue to create nanostructured metal oxide/graphene materials for advanced battery applications. For lithium-ion batteries (LIBs), the cathode is typically a metal oxide and serves as the host for Li + ion intercalation during the charge/discharge process. Different metal oxides have been explored as cathode materials [1] . Among the commonly used cathode materials such as LiCoO 2 (274 mAh g −1 ) [2] and LiFePO 4 (170 mAh g −1 ) [3] , vanadium pentoxide (V 2 O 5 ) has a theoretical capacity of 443 mAh g −1 (assuming intercalation of three lithium ions) and a specific energy of 1,218 mWh g −1 (assuming a nominal 2.75 V discharge voltage). In addition, vanadium is abundant in the crust of the earth, which makes it inexpensive. The combination of the high specific capacity/energy and its abundance make V 2 O 5 a very attractive candidate for LIB applications. However, the high specific capacity/energy has not been realized in practical LIB applications [4] , [5] , [6] , [7] , [8] , [9] , [10] because of these three issues: (1) low electrical conduction, (2) slow lithium-ion diffusion and (3) irreversible phase transitions upon deep discharge. Like most metal oxides, V 2 O 5 has very low electronic conductivity due to its low d -band mobility [11] . The lithiation/delithiation processes in crystalline V 2 O 5 are accompanied by structural phase transitions [12] . Such a phase transition process induces lattice strain due to phase coexistence within the same electrode particle. It is known that the lattice mismatch-induced mechanical strain can cause irreversible structural damage, which not only limits battery life, but also causes irreversible capacity loss [13] . Consequently, V 2 O 5 currently has very poor rate capability and very limited long-term cyclability. Compared with crystalline V 2 O 5 , the amorphous V 2 O 5 xerogel offers a considerable advantage by virtue of its morphology. The vanadium oxide xerogel, V 2 O 5 ·nH 2 O has a ribbon-like structure, providing more access for Li + ion insertion than its crystalline counterpart, leading to a more versatile host for Li + ion intercalation and exhibiting improved capacity for the lithium [14] . The basic units of the V 2 O 5 xerogel are sheets comprised of two vanadium oxide layers [1] . When the distance of the adjacent layers of V 2 O 5 increases, the insertion capacity will increase. Hence, in hydrated V 2 O 5 xerogel, V 2 O 5 ·nH 2 O, the water molecules function as pillars between the V 2 O 5 layers and support a basal spacing of ~11.5 Å [15] , leading to a Li intercalation capacity about 1.4 times larger than that of orthorhombic V 2 O 5 ,(~4.56 Å). In addition, the larger interlayer spacing also facilitates the Li + diffusion within the V 2 O 5 matrix [16] . In addition, the interlayered water molecules result in a distorted square–pyramidal ligand field that favours electron transfer and Li + intercalation within the V 2 O 5 matrix [16] . However, even for V 2 O 5 xerogel, the same challenges of low electrical conduction (both intraparticle, within a V 2 O 5 particle, and interparticle, between V 2 O 5 particles), slow lithium diffusion and structure stability/reversibility still remain. Efforts have been made to improve the conductivity by coating the V 2 O 5 xerogel with conductive materials (that is, single-wall carbon nanotubes) [17] , doping metals [18] and organic polymers [19] , [20] , [21] , [22] , [23] . These measures can improve the V 2 O 5 xerogel only to a certain degree, and none of them significantly improve the structural stability and reversibility. Hence, a comprehensive approach that can simultaneously deal with all three of these issues is needed. Graphene is a single-atomic layer of sp 2 -bonded carbon atoms arranged in a honeycomb crystal structure [24] , which provides extraordinary electrical (that is, extremely high electric conductivity—6.29*10 7 S cm −1 ), mechanical (that is, fracture strength ~130 GPa) and thermal properties (that is, 3,000 W/m-K in plane) [25] . Graphene can be prepared using either the chemical or thermal reduction of graphene oxide (GO), which is a layered stack of oxidized graphene sheets with different functional groups. Thus, GO can be easily dispersed in the form of a single sheet in water at low concentrations. Our comprehensive approach for dealing with these three issues of the V 2 O 5 xerogel is to insert a single graphene sheet to, at most, a few layers of graphene sheets between the V 2 O 5 nanoribbons to modify the V 2 O 5 xerogel structure via the sol–gel process. Such a structure can be expected to improve both the intraparticle electronic conduction and the lithium-ion diffusion. Furthermore, the resulting smaller V 2 O 5 grain size in the V 2 O 5 xerogel can be expected to reduce the stress within the particles, leading to better structural stability and cycle life. Here we report a simple and unique method for synthesizing graphene-modified, nanostructured V 2 O 5 via the sol–gel process, leading to the creation of a class of V 2 O 5 hybrids with intercalated graphene at low concentrations (that is, 2 wt. %). We demonstrate that these V 2 O 5 /graphene hybrid materials have overcome the above-mentioned three major issues and exhibit extraordinary electrochemical performance as cathode materials for LIBs. In operando synchrotron high-energy X-ray diffraction (HEXRD), X-ray absorption near-edge spectroscopy (XANES), cryo-transmission electron microscopy (cryo-TEM) and low-voltage, aberration-corrected high-resolution TEM are used to characterize their structure and to elucidate the formation mechanism of these materials, providing a foundation for understanding their extraordinary performance. Electrochemical performance The introduction of a tiny amount of graphene (that is, 2 wt. %) into the V 2 O 5 has an extraordinary effect on its electrochemical performance. In the following discussion, we define the graphene-modified nanostructure–V 2 O 5 hybrid as ‘V 2 O 5 –G’ and V 2 O 5 without graphene as ‘pure V 2 O 5 ’. A specific capacity of 438 mAh g −1 (corresponding to 1,034 Wh kg −1 and 3,118 Wh l −1 ) has been achieved at 0.05 C ( Fig. 1a ) for the V 2 O 5 –G with 2% graphene, which is almost to the theoretical specific capacity, 99% of 443 mAh g −1 (theoretical value), while the pure V 2 O 5 delivered only 324 mAh g −1 (corresponding to 777 Wh kg −1 ). The achieved 438 mAh g −1 also suggests that the three Li + ions have been reversibly inserted/de-inserted into each V 2 O 5 molecule in the V 2 O 5 –G hybrid. In addition to the high specific capacity, this V 2 O 5 –G hybrid shows the excellent reversibility (of capacity) from the voltage profile, which indicates that most of the inserted lithium ions can be removed during the discharge/charge process. Even at a higher rate, 1 C, such V 2 O 5 –G still delivered 315 mAh g −1 (corresponding to 768 Wh kg −1 ; Fig. 1b ), which is 2.23 times that of the pure V 2 O 5 , 137 mAh g −1 (corresponding to 299 Wh kg −1 ). The pure V 2 O 5 discharge profile shows three distinct voltage stages: 3.3-2.5 V, 2.5-2.0 V and 2.0-1.75 V, corresponding to the first, second and third Li + ion intercalations into the V 2 O 5 ( Fig. 1b ). However, no such voltage plateaus were seen for the V 2 O 5 –G, which is typical for a disordered layer or single-phase material due to the absence of the crystalline phase transitions [26] . It is expected that the lower crystallinity should lead to less stress on the material and better cycle performance. 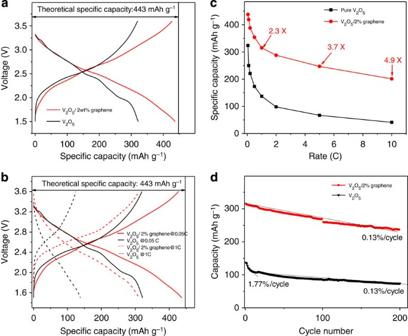Figure 1: Electrochemical characterization. Charge/discharge curves of pure V2O5and V2O5–G/2% graphene cells at (a) 0.05 and (b) 0.05 and 1.0 C; (c) rate performance of pure V2O5and V2O5–G/2% graphene cells based on C-rate and (d) cycle life of pure V2O5and V2O5–G with 2% graphene cells at a 1 C rate. Figure 1: Electrochemical characterization. Charge/discharge curves of pure V 2 O 5 and V 2 O 5 –G/2% graphene cells at ( a ) 0.05 and ( b ) 0.05 and 1.0 C; ( c ) rate performance of pure V 2 O 5 and V 2 O 5 –G/2% graphene cells based on C-rate and ( d ) cycle life of pure V 2 O 5 and V 2 O 5 –G with 2% graphene cells at a 1 C rate. Full size image The introduction of graphene also has a significant effect on the rate performance, which is a major issue for pure V 2 O 5 . At fairly higher current densities, the V 2 O 5 –G still retains a high capacity: 419 mAh g −1 at 0.1 C, 354 mAh g −1 at 0.5 C, 315 mAh g −1 at 1 C, 247 mAh g −1 at 5 C and 201 mAh g −1 at 10 C, as compared with those of pure V 2 O 5 : 250 mAh g −1 at 0.1 C, 173 mAh g −1 at 0.5 C, 137 mAh g −1 at 1 C, 67 mAh g −1 at 5 C and 41 mAh g −1 at 10 C ( Fig. 1c ). This corresponds to a 67.6, 104.6, 130.0, 268.7 and 390.2% specific capacity increase at the different rates, respectively. Such a huge improvement on rate performance, particularly at high rates (that is, 10 C), suggests that it not only has the electric conductivity of the V 2 O 5 –G tremendously increased (both interparticle and intraparticle conductivity), but also that the ionic conductivities have increased. This is clearly seen from the alternating current (AC) impedance data, shown in Fig. 2 and described in detail below. 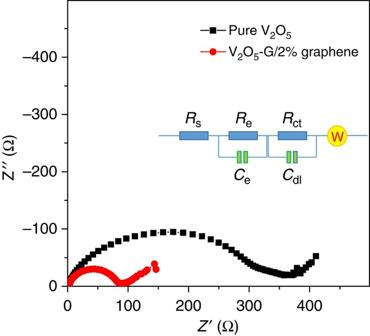Figure 2: Electrochemical impedance spectroscopy (Nyquist plot). Electrochemical impedance spectroscopy (Nyquist plot) of the pure V2O5and the V2O5–G/2% graphene cells. Amplitude: 5 mV, frequency range: 1 MHz–0.01 Hz Figure 2: Electrochemical impedance spectroscopy (Nyquist plot). Electrochemical impedance spectroscopy (Nyquist plot) of the pure V 2 O 5 and the V 2 O 5 –G/2% graphene cells. Amplitude: 5 mV, frequency range: 1 MHz–0.01 Hz Full size image The synthesized V 2 O 5 –G also exhibits improved cycling stability. The V 2 O 5 –G achieved 150 cycles with 80% initial capacity at a 1 C rate, while the pure V 2 O 5 achieved only 11 cycles ( Fig. 1d ). (The death criteria of a battery for electric vehicle and hybrid electric vehicle is defined as 80% of its initial capacity; hence, we compare the cycle life at 80% initial capacity.) The capacity decay rate is relatively stable for V 2 O 5 –G, at 0.13%/cycle, while the pure V 2 O 5 shows two distinctly different decay rates: it initially decays sharply at 1.77%/cycle to 80% initial capacity after 11 cycles; after 12 cycles, it decays at a much slower rate of 0.13%/cycle, indicating that the pure V 2 O 5 might experience a structure change during the initial cycles and that then the structure becomes stabilized. The content of graphene in the V 2 O 5 –G plays a critical role. Clearly, 2% graphene results in the highest specific capacity, 438 mAh g −1 ( Supplementary Fig. 1 ), while 10% graphene leads to a lower specific capacity, 278 mAh g −1 , but much improved cycle stability. It is speculated that the lower graphene content may result in a better dispersion of the graphene sheets in the hydrogel of the V 2 O 5 , while the higher graphene content may lead to the restacking of the graphene sheets, as we observed in our previous work [27] . The thicker stacks of graphene (that is, 3–5 graphene sheets per stack) may hold the V 2 O 5 nanoribbons tighter and, thus, help maintain the structural integrity, consequently leading to a much better cycle life. Another possibility is that the higher graphene content may lead to more complete coverage over the V 2 O 5 nanoribbons, which could help to hold the ribbons together and prevent them from collapsing. A detailed understanding of the effects of the graphene content in the V 2 O 5 –G is another topic of study and will be reported separately. AC impedance spectra of both pure V 2 O 5 and V 2 O 5 –G were measured to validate that our approach of inserting the graphene sheets between the V 2 O 5 nanoribbons via the sol–gel process leads to improved electric conductivity, Li + ion diffusion and structural stability. The results were fitted using the model [28] shown in Fig. 2 , and the fitting results are listed in Supplementary Table 1 . Clearly, the small amount of graphene in the V 2 O 5 caused a huge change in the electric conductivity, R e , from 309.48 Ω in pure V 2 O 5 to 86.55 Ω in V 2 O 5 –G, an order of magnitude change. Both the pure V 2 O 5 and the V 2 O 5 –G electrodes had the exact same composition and were made using the same procedures under the same conditions; therefore, the change in the R e must be due to the conductivity of V 2 O 5 . This is similar to the doping of Cu into the V 2 O 5 xerogel by Symerl et al . [18] The redox reaction of vanadium in the V 2 O 5 also increased significantly. The R ct changed from 46.88 Ω in the pure V 2 O 5 to 10.94 Ω in the V 2 O 5 –G. This is a 4.28X change that also explains the increased rate performance. Finally, the Li + ion diffusion within the V 2 O 5 has improved. The W d changed from 0.451 to 0.396, corresponding to a Li + diffusion coefficient in the V 2 O 5 that changed from 1.21 E−12 to 1.57 E−12 cm 2 s −1 , a 12% increase. Thus, the AC impedance results show that our approach, indeed, works as we designed. From the data, it is clear that the introduction of a small amount (that is, 2%) of graphene has a profound effect on the electrochemical performance of V 2 O 5 , and the V 2 O 5 –G shows the best electrochemical performance of any reported V 2 O 5 hybrids in the coin cell configuration, as summarized in Supplementary Table 2 (refs 5 , 7 , 29 , 30 , 31 , 32 , 33 , 34 , 35 , 36 , 37 , 38 , 39 , 40 , 41 , 42 , 43 ). However, all performance changes are rooted in the material structure. Hence, in operando XANES, in operando HEXRD, cryo-TEM and aberration-corrected TEM were carried out to understand the structure and the formation mechanisms of the V 2 O 5 –G. The results are presented below. Formation mechanism and morphology of pure V 2 O 5 and V 2 O 5 –G As demonstrated previously, the introduction of a small amount of graphene can cause a huge performance change for the formed V 2 O 5 –G. Naturally, a question arises: how could such a small amount of graphene (~2% weight) change the structure of the V 2 O 5 xerogel? Aiming to understand the effects of graphene on the structure of the V 2 O 5 xerogel, the synthesis process of V 2 O 5 –G was studied using cryo-TEM. As described below, sodium metavanadate (NaVO 3 ) becomes yellow coloured decavanadic acid (HVO 3 ) after passing through an ion exchange column. This diluted HVO 3 starts to slowly form a V 2 O 5 hydrogel via the protonation of HVO 3 (usually within several minutes) [23] ; the solution gradually changes colour from yellow to dark brown and, eventually (usually after 1–2 weeks), to dark red, indicating the completion of the formation of a three-dimensional network of V 2 O 5 hydrogel. The 3.5 μl aliquots of HVO 3 solution were taken at 0, 30, 45, 60, 90, 120, 360 min and 1, 2 and 3 weeks to monitor the process of initializing, nucleating and growing the ribbons for the V 2 O 5 xerogel (the time at 0 min refers to the time when about 5 ml of the HVO 3 solution came out from the ion exchange column). The advantage of cryo-TEM is that it can directly observe the microgeometry and the morphology of particles within a liquid without disturbance by fast freezing the liquid sample using liquid N 2 , which preserves the morphology and microgeometry of the particles in the original liquid. We have successfully used cryo-TEM in our previous work to perform similar characterizations [44] . The nucleation immediately (0 min) occurred once the HVO 3 solution was formed (right after NaVO 3 passed through the ion exchange column) ( Fig. 3a ). Then, small V 2 O 5 ribbons started to grow into 100 nm long ribbons with diameters of a few nanometres, as shown in the 60-min image ( Fig. 3b ). The V 2 O 5 ribbons grew more rapidly in one direction, with the shorter dimension never growing larger than those observed after 90 min ( Fig. 3c ). Finally, after 2 weeks, the V 2 O 5 hydrogel network was formed with a similar length but much larger width than the V 2 O 5 ribbons ( Fig. 3d ). It is very interesting to see that when the GO was added into the HVO 3 solution, the V 2 O 5 hydrogel formation took place on the surface of the GO sheets. First, the solution nucleated, small ribbons formed, the ribbons grew and finally, the V 2 O 5 hydrogel network formed. On adding the GO solution into the HVO 3 solution, the nuclei that formed in the beginning tended to adsorb on the GO sheets due to the Coulombic interaction and van der Waals force between the nuclei and the GO. 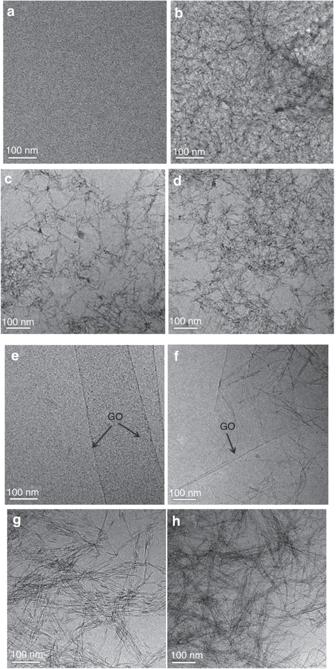Figure 3: Cyro-TEM images of the frozen solution during different aging processes. For pure HVO3: (a) nucleation (0 min), (b) vanadium oxide ribbon growth (1 h), (c) continuous growth of V2O5ribbons (1 h 30 min.) and (d) fully grown vanadium oxide ribbons (2 weeks). For the mixture of HVO3and the GO solution: (e) nucleation (30 min), (f) vanadium oxide ribbon growth (2 h), (g) continuous growth of V2O5ribbons (6 h) and (h) fully grown vanadium oxide ribbons (3 weeks) Figure 3: Cyro-TEM images of the frozen solution during different aging processes. For pure HVO3: ( a ) nucleation (0 min), ( b ) vanadium oxide ribbon growth (1 h), ( c ) continuous growth of V 2 O 5 ribbons (1 h 30 min.) and ( d ) fully grown vanadium oxide ribbons (2 weeks). For the mixture of HVO 3 and the GO solution: ( e ) nucleation (30 min), ( f ) vanadium oxide ribbon growth (2 h), ( g ) continuous growth of V 2 O 5 ribbons (6 h) and ( h ) fully grown vanadium oxide ribbons (3 weeks) Full size image In contrast to pure V 2 O 5 , the nucleation of the V 2 O 5 hydrogel in the presence of GO sheets took a much longer time: after 30 min, the nucleation started ( Fig. 3e ), which probably was due to the repulsive effect from some regions of the GO surface having negative charges for the different functional groups (that is, phenol, carbonyl, ketone, etc.) [45] . After 120 min, very few pieces of the V 2 O 5 ribbons could be seen ( Fig. 3f ). Even after 6 h, the V 2 O 5 ribbons continuously grew, but with much lower density than pure V 2 O 5 ( Fig. 3g ). Finally, it took 3 weeks to form the fully grown V 2 O 5 hydrogel network ( Fig. 3h ). However, the V 2 O 5 ribbons in the fully grown V 2 O 5 hydrogel on the GO surface looked more uniform, had a much smaller range of width, and were much less densely arranged than the pure V 2 O 5 hydrogel (compared in Fig. 3d,h ). This must be attributed to the existence of the GO sheets, which provides a substrate for the V 2 O 5 hydrogel formation but at a much slower rate. It appears that this facilitates crystal growth rather than nucleation due to the negative charge repulsion. Thus, the V 2 O 5 ribbons are formed with a smaller width and are much less densely arranged over the GO surface. This leads to the smaller grain size of the V 2 O 5 ribbons, which correlates to improved Li + diffusion as indicated by AC impedance results and to reduced lattice stress as evidenced by the increased cycle life. The less densely arranged V 2 O 5 ribbons over the GO surface also result in more gaps between the V 2 O 5 ribbons, providing more surface area for Li + diffusion into the ribbons. Clearly, the graphene sheets serve as a substrate for the V 2 O 5 ribbons and lead to the tremendous increase in electric conductivity. On the other hand, the V 2 O 5 formation over the GO surface requires that the V 2 O 5 anchor on the GO first, which makes the overall V 2 O 5 ribbon formation take a much longer time than it does in the liquid. This GO-aiding synthesis led to a uniform distribution of the GO sheets within the V 2 O 5 nanoribbons, as evidenced by the scanning electron microscopy images and energy-dispersive X-ray spectroscopy mapping ( Supplementary Fig. 2 ). The proposed synthesis scheme of a V 2 O 5 /GO hybrid is shown in Fig. 4 , and, for clarity, only the V 2 O 5 on one side of the GO sheet was drawn. As the GO is a single layer, the GO sheets act as spacers to create gaps between the formed V 2 O 5 nanoribbons once the water is removed from the V 2 O 5 hydrogel by heating. In other words, the V 2 O 5 nanoribbons may be sandwiched between the layers of graphene after annealing. Such V 2 O 5 nanoribbons with a 5–10 nm diameter were anchored or sandwiched between the graphene sheets, as clearly seen in Fig. 5a (indicated by the yellow dashed circle region). In addition, a low-voltage, aberration-corrected high-resolution TEM image of the synthesized V 2 O 5 –G in Fig. 5b clearly shows the V 2 O 5 nanoribbons sandwiched in between the graphene sheets. The electron energy loss spectroscopy (EELS) data ( Supplementary Fig. 3 ) shows that the oxidation state of vanadium in the V 2 O 5 –G hybrid remained unchanged, indicating that the intercalation of the GO/graphene sheets into the V 2 O 5 layers did not cause the change in the oxidation state of the vanadium. 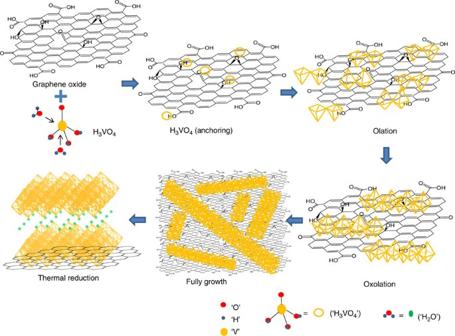Figure 4: A proposed synthesis scheme of V2O5/graphene hybrids. Olation: each VO(OH)3(OH)2molecule is bridged by OH group to form a polymer chain; oxolation: slower oxolation reactions convert unstable 2(OH)1 (2(OH)1 repents a OH group bridges two VO(OH)3(OH2)2molecules) into stable 3(O)1 bridges (an oxygen connects three VO(OH)3(OH2)2molecules, forming double chains). Further oxolation involving the last OH groups link these double chains together so that V2O5nanofibres formed Figure 4: A proposed synthesis scheme of V 2 O 5 /graphene hybrids. Olation: each VO(OH) 3 (OH) 2 molecule is bridged by OH group to form a polymer chain; oxolation: slower oxolation reactions convert unstable 2(OH)1 (2(OH)1 repents a OH group bridges two VO(OH) 3 (OH2) 2 molecules) into stable 3(O)1 bridges (an oxygen connects three VO(OH) 3 (OH2) 2 molecules, forming double chains). 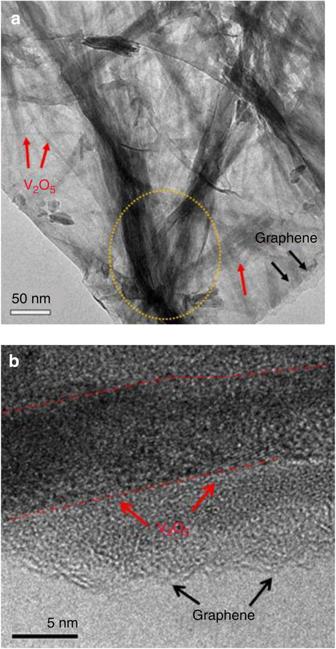Figure 5: TEM characterization of the V2O5–G hybrids. (a) TEM of as-synthesized V2O5–G hybrid after calcination. (Note: in panels, the black arrows point to the graphene sheets, the red arrows point to the V2O5nanoribbons and the yellow dashed circle points out the area where the graphene and nanoribbons twist together.). (b) HRTEM of as-synthesized V2O5–G hybrid after calcination. (Note: the red dashed line points out the area where a V2O5nanoribbon is located). Further oxolation involving the last OH groups link these double chains together so that V 2 O 5 nanofibres formed Full size image Figure 5: TEM characterization of the V 2 O 5 –G hybrids. ( a ) TEM of as-synthesized V 2 O 5 –G hybrid after calcination. (Note: in panels, the black arrows point to the graphene sheets, the red arrows point to the V 2 O 5 nanoribbons and the yellow dashed circle points out the area where the graphene and nanoribbons twist together.). ( b ) HRTEM of as-synthesized V 2 O 5 –G hybrid after calcination. (Note: the red dashed line points out the area where a V 2 O 5 nanoribbon is located). Full size image In operando HEXRD characterization of V 2 O 5 –G To further understand the structure of V 2 O 5 –G, in operando HEXRD was measured for both V 2 O 5 –G and pure V 2 O 5 during the heating process. The results for pure V 2 O 5 are shown in Fig. 6a . Initially, the sample showed the layered hydrated V 2 O 5 ( 00l ) reflections, a typical disordered layer structure. The layered structure was maintained until about 200 °C; then, the ( 00l ) reflection shifted slowly to a higher 2-theta angle. The shift was primarily caused by the loss of water molecules between the V 2 O 5 layers [16] , resulting in the shortening of the interlayer spacing between the V 2 O 5 layers. The transition from the disordered layer phase to the crystalline phase started around 200 °C, ( Fig. 6a ; inset): the newly emerged peak, around 1.42°, is attributed to the orthorhombic V 2 O 5 (JCPDS No, 41-1426). The loss of water from in between the V 2 O 5 layers correlates with the observed phase transformation. As the temperature continued to increase, the peak intensity of the crystalline V 2 O 5 rapidly increased at the expense of the relative peak intensity of the layer hydrated structure (amorphous). Finally, at around 400 °C, the amorphous phase almost completely diminished and the phase transformation was completed. The V 2 O 5 xerogel structure collapsed due to the complete removal of crystal water from the V 2 O 5 on heating to 400 °C; then, the V 2 O 5 xerogel completely transformed into a V 2 O 5 nanocrystal, which shows three distinct discharge stages ( Fig. 1a,b ). 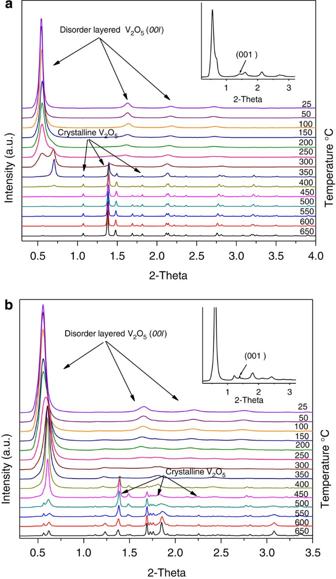Figure 6:In operandoHEXRD characterization of pure V2O5and V2O5–G. (a) XRD patterns of the V2O5xerogel during the heat treatment process between room temperature and 600 °C, showing that the bi-pyramid structure completely collapses at around 400 °C and (b) XRD patterns of V2O5–G with graphene during the heat treatment process between room temperature and 600 °C, showing that the bi-pyramid structure persists until 450 °C Figure 6: In operando HEXRD characterization of pure V 2 O 5 and V 2 O 5 –G. ( a ) XRD patterns of the V 2 O 5 xerogel during the heat treatment process between room temperature and 600 °C, showing that the bi-pyramid structure completely collapses at around 400 °C and ( b ) XRD patterns of V2O5–G with graphene during the heat treatment process between room temperature and 600 °C, showing that the bi-pyramid structure persists until 450 °C Full size image It is interesting to note that the graphene had a significant impact on the structure of the V 2 O 5 hybrid. Initially, the V 2 O 5 –G showed a layered hydrated structure similar to that of pure V 2 O 5 but with larger interlayer spacing ( d -spacing), indicating that the intercalation of the GO sheets leads to increased interlayer spacing between the V 2 O 5 layers. At room temperature, the d -spacing of the V 2 O 5 –G is about 13.65 Å, which is much higher than that of the pure V 2 O 5 , 11.40 Å. Similar XRD results on the intercalation of polymers between V 2 O 5 layers in xerogel have been observed, suggesting that the interlayer spacing increased to between ~12.0 and ~15.0 Å, depending on the type of the polymer [46] , [47] , [48] , [49] . As the temperature increased, the ( 00l ) reflection shifted to a higher 2-theta angle in a manner similar to that of the pure V 2 O 5 sample, but at a much slower rate. Unlike the pure V 2 O 5 , which transitioned from the disordered layer phase to the crystal phase starting around 200 °C, the phase transition for V 2 O 5 –G started around 400 °C as indicated by the emerging peak at 1.42° ( Fig. 6b ). Clearly, with the presence of graphene, the disordered-to-crystalline phase transition was delayed. Obviously, in analogy to the pure V 2 O 5 , for the hybrid, the thermal stability will be greatly enhanced when the V 2 O 5 layer is affixed to the graphene sheets. For the electrochemical performance testing, the obtained V 2 O 5 –G was annealed at 400 °C in N 2 before being used as the cathode. The HEXRD data in Fig. 6b show that the calculated V 2 O 5 interlayer spacing, d -spacing, was 10.2 Å, corresponding to 0.3 water per V 2 O 5 , V 2 O 5 ·0.3H 2 O (refs 8 , 16 ). However, for the pure V 2 O 5 , there was almost no water left at 400 °C and the structure completely changed to a nanocrystal instead of the layered V 2 O 5 xerogel. Crystallized water inside the V 2 O 5 xerogel functions as ‘pillars’ to keep the interlayer spacing fixed between the two V 2 O 5 sheets. For the V 2 O 5 xerogel, the large amount of water may react with the lithium to form Li 2 O, which deteriorates intercalation performance [8] . Without water molecules to act as the pillars, the V 2 O 5 network in the disordered layer V 2 O 5 xerogel will collapse during annealing and become crystalline V 2 O 5 , which has much lower electrochemical performance. Hence, a minimum amount of crystal water is needed to keep the disordered layer phase. Thus, the graphene-sheet-modified V 2 O 5 layers do increase the thermal stability and preserve the disordered layer phase even at 400 °C with 0.3 water per V 2 O 5 . Thermogravimetric analysis (TGA) was also carried out for both pure V 2 O 5 and V 2 O 5 –G to study the structure change during annealing, and the results are shown in Fig. 7 . The pure V 2 O 5 xerogel had a rapid weight loss (0.15%/°C) until 80 °C, followed by a gradual weight loss at a much slower rate (0.018%/°C) up to 300 °C, which corresponds to the loss of weakly bonded water molecules in the V 2 O 5 xerogel [23] . As temperatures went to beyond 200 °C, the tightly bonded water molecules—crystallized water molecules—were removed, and the phase conversion from the disordered layer phase to the orthorhombic phase started [16] . This is consistent with our HEXRD results. Compared with the pure V 2 O 5 , the V 2 O 5 –G showed a completely different profile; it had a gradual weight loss at a rate of 0.024%/°C until 250 °C, which is characteristic of the loss of weakly bonded water from the V 2 O 5 –G. This was followed by another gradual weight loss with a slightly faster slope (0.05%/°C) until 450 °C. In terms of the crystal structure, the bi-pyramid structure persisted below 450 °C, although there were indications of the nucleation of the orthorhombic V 2 O 5 phase at around 400 °C. The TGA results further verified that the thermal stability of the V 2 O 5 was greatly enhanced by the presence of graphene. 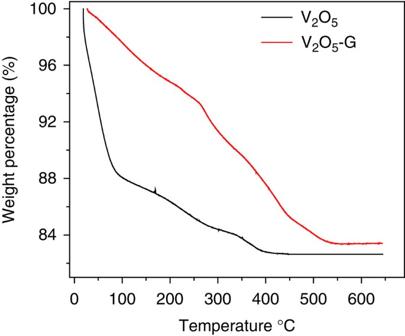Figure 7: Thermogravimetric analysis. Comparison of TGA curves between pure V2O5xerogel and V2O5–G. Figure 7: Thermogravimetric analysis. Comparison of TGA curves between pure V 2 O 5 xerogel and V 2 O 5 –G. Full size image In operando XANES analysis In operando XANES characterization of V 2 O 5 –G during the electrochemical process was carried out at 20-BM-B, Advanced Photon Source. The two-dimensional (2D) contour plots of in operando XANES spectra for the V 2 O 5 –G are shown in Fig. 8a . In addition, the voltage profile is displayed on the side of the XANES data for comparison. Obviously, the electrochemical process correlates well with the evolution of the XANES data. Typical vanadium XANES during the first discharge process is shown in Fig. 8b and illustrates the insertion of lithium ions into the V 2 O 5 –G. On the insertion of the lithium ions, the K-edge of the vanadium continuously shifted towards the lower binding energy. This shift indicates a decrease in the average valence state of vanadium, which corresponds to the increase in the number of inserted Li + ions in each V 2 O 5 . At the fully discharged state, the emerging shoulder (labelled by the an arrow) was found, which is consistent with the reduction of V(IV) to V(III) [50] . During the charge process after the first discharge, the K-edge of the vanadium shifted towards the higher binding energy ( Supplementary Fig. 4 ). 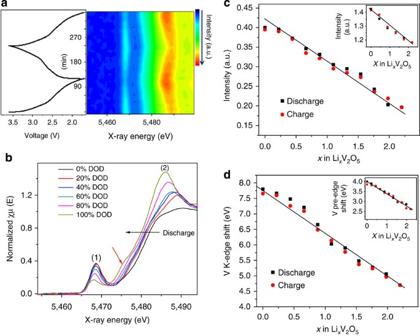Figure 8: In operando XANES characterization of the Li/V2O5–G coin cells during discharge/charge cycling. (a) Normalized XANES spectra (2D contour plot) and voltage profiles of Li/V2O5–G coin cells during cycling. (b) Typical vanadium K-edge XANES spectra during the first discharge process. (c) XANES pre-edge peak and main peak (inset) intensities as a function of lithium composition during the first charge/discharge process. (d) V K-edge energy (at half weight) shift and pre-edge shift (inset) as a function of lithium composition during the first charge/discharge process. The Li content for the lithiated samples (that is,xin LixV2O5) was calculated from the electrochemical results. The energy shift uses vanadium as the reference Figure 8: In operando XANES characterization of the Li/V 2 O 5 –G coin cells during discharge/charge cycling. ( a ) Normalized XANES spectra (2D contour plot) and voltage profiles of Li/V 2 O 5 –G coin cells during cycling. ( b ) Typical vanadium K-edge XANES spectra during the first discharge process. ( c ) XANES pre-edge peak and main peak (inset) intensities as a function of lithium composition during the first charge/discharge process. ( d ) V K-edge energy (at half weight) shift and pre-edge shift (inset) as a function of lithium composition during the first charge/discharge process. The Li content for the lithiated samples (that is, x in Li x V 2 O 5 ) was calculated from the electrochemical results. The energy shift uses vanadium as the reference Full size image Besides the K-edge, there are two other important features in the XANES region: the pre-edge (labelled 1 in Fig. 8b ) and the edge resonance (labelled 2 in Fig. 8b ), which are also sensitive to the valence state of the vanadium and the chemical environment surrounding the vanadium site [51] . As the intensity of the pre-edge peak was consistent with the deviation from the octahedral symmetry of the vanadium site [52] , the intensity of the pre-edge decreased and the peak ‘1’ position shifted towards the lower energy during the discharge process ( Fig. 8b ). The edge resonance, which is related to the energy absorption by core electrons, showed major changes in both intensity and shape [53] . During the discharge process, the shape changed from two well-defined peaks to a single peak (peak ‘2’ in Fig. 8b ) and the intensity increased, while during the charge process, the intensity decreased and the shape changed from a single peak back to two well-defined peaks ( Supplementary Fig. 4 ). A similar reversible behaviour for the pre-edge, the edge and the edge resonance was also observed by Smyrl et al . [54] on V 2 O 5 xerogel cathodes. To further establish the intensity change and energy shift of the pre-edge, the edge and the edge resonance, a combined Gaussian-arctangent fit was performed [55] , and the results are shown in Fig. 8c . As discussed earlier, the V 2 O 5 gel-based materials consist of distorted, square-based pyramids with four basal oxygen atoms and one apical oxygen atom [1] . The intensity of the pre-edge directly correlates to the distortion of the V 2 O 5 square pyramid, while the intensity of the edge resonance is associated with the symmetry of the basal oxygen configuration around the vanadium site [53] . Obviously, the intensity of the pre-edge peak and the edge resonance ( Fig. 8c , inset) peak showed major changes but exhibited a linear decrease. Importantly, the intensities during the charging process also changed linearly, which confirms the structural reversibility of the hybrid. The XANES K-edge and pre-edge shift as a function of Li composition in the V 2 O 5 –G is shown in Fig. 8d . Obviously, both the K-edge and pre-edge energy shifts ( Fig. 8d , inset) varied linearly with the valence of the vanadium atom. Importantly, the energy shifts during the charge process also showed a linear change, which confirms the electronic reversibility of the hybrid. In summary, our in operando XANES measurements clearly reveal the electronic and structural reversibility of the V 2 O 5 –G during the lithium insertion and de-insertion process. On the other hand, the excellent performance of the V 2 O 5 –G can be ascribed to the reversibility of the intercalation process and preserved single phase of the composite, as can be seen in the in operando HEXRD results ( Fig. 6b ). Compared with the crystalline V 2 O 5 , the stabilized layered structure will undoubtedly allow easier lattice expansion and contraction during the discharge/charge process without any major distortion of the V 2 O 5 hybrid structure. To date, graphene has been considered an ideal conducting material to improve the electrical conductivity and enhance the structure of V 2 O 5 [10] , [43] , [56] , [57] . However, most composites have been created by simply mixing graphene with the V 2 O 5 . Such simple physical mixing usually requires high graphene loadings (for example, 30% graphene [56] ), which leads to a significant improvement on the cycle life and rate performance, but with a heavy penalty on the specific capacity. In this work, a method of creating V 2 O 5 –G via the sol–gel process has been developed, and we have demonstrated that although a small amount of graphene is used, there is a profound effect on the structure. This structural change consequently results in extraordinary electrochemical performance without a heavy penalty on specific capacity; in fact, the material nearly achieves the theoretical specific capacity. We clearly demonstrated through our in operando HEXRD that the graphene sheets help to preserve the V 2 O 5 layered structure and keep the xerogel from collapsing to form the orthorhombic crystalline phase during the annealing process. In addition, the AC impedance proves that the electric conductivity, the vanadium redox reaction and the Li + diffusion have been improved due to the introduction of such a small amount of graphene. The performance of electrode materials is always rooted in the materials structure [58] , [59] . The graphene sheets sandwiched in between the V 2 O 5 layers not only enhance the electron conduction between the V 2 O 5 layers (intraparticle conduction, supported by TEM and XRD results) and between the V 2 O 5 ribbons (inter-particles conduction, supported by Cryo-TEM results), but also preserve the water molecules between the two layers of V 2 O 5 , which facilitates the Li + diffusion (as can be seen from the AC impedance results). The combined effect on electronic conduction and Li + diffusion significantly improves the electrochemical performance. Furthermore, the presence of the graphene sheets between the V 2 O 5 layers enhances the structural integrity of the disordered V 2 O 5 –G during cycling, resulting in the improved reversibility of the intercalation process and in the preserved single phase of the hybrid composite, which in turn, leads to a significantly improved cycle life. In summary, we have demonstrated a novel and simple method to incorporate graphene sheets into the nanostructure of V 2 O 5 xerogel via a sol–gel process, forming a graphene-modified V 2 O 5 hybrid with a stabilized layered structure. The reversible charge/discharge of 438 mAh g −1 capacity indicated that the three Li + ions have been successfully inserted/desinserted to the V 2 O 5 /graphene hybrid. The introduction of a small amount of graphene into the V 2 O 5 can effectively alter the structure of the nanocomposite, resulting in significant improvements in electric conductivity, structural stability and ion diffusion. This, in turn, results in extraordinary electrochemical performance of the graphene-modified V 2 O 5 hybrid. The hybrid nearly reached the theoretical specific capacity and demonstrated excellent rate performance and greatly enhanced cycle life. This method provides a new avenue to create nanostructured materials with improved properties for metal oxides as long as they can be synthesized via the sol–gel process or by a reaction in a solution. The sol–gel process and the solution method are both easy for scale-up, and the starting materials are abundant, which makes widespread industrial application of these new materials feasible. Synthesis of V 2 O 5 xerogel The V 2 O 5 xerogel was prepared by a simple, modified ion exchange method [23] , [48] , [60] , [61] . A 0.1 M solution of NaVO 3 (Sigma, >99.5%) was eluted through a column loaded with a proton-exchange resin (Dowex-50-WX2, 50–100 mesh). The obtained yellow solution of HVO 3 was aged in a glass container for 2 weeks to obtain a mature homogeneous vanadium oxide hydrogel. Dried xerogel was obtained by freeze drying the hydrogel under vacuum. Synthesis of GO GO was prepared using two methods. First, 2 g of graphite flakes were mixed with 10 ml of concentrated H 2 SO 4 , 2 g of K 2 S 2 O 8 and 2 g of P 2 O 5 . The obtained mixture was heated at 80 °C for 4 h with constant stirring. Then the mixture was filtered and washed thoroughly with deionized (DI) water. After drying in an oven at 80 °C overnight, this pre-oxidized graphite was then subjected to oxidation using Hummer’s method [45] . Next, 2 g of pre-oxidized graphite, 1 g of sodium nitrate and 46 ml of sulfuric acid were mixed and stirred for 15 min in an ice bath. Then, 6 g of potassium permanganate was slowly added to the obtained suspension solution for another 15 min. After that, 92 ml DI water was slowly added to the suspension, while the temperature was kept constant at about 98 °C for 15 min. After the suspension was diluted by 280 ml DI water, 10 ml of 30% H 2 O 2 was added to reduce the unreacted permanganate. Finally, the resulting suspension was centrifuged several times to remove the unreacted acids and salts. The purified GO was dispersed in DI water by sonication for 1 h to form a 0.2 mg ml −1 solution. Then the GO dispersion was subjected to another centrifugation to remove the un-exfoliated GO. The resulting GO diluted solution could remain a very stable suspension without any precipitation for a few months [27] . Synthesis of a graphene-modified nanostructured V 2 O 5 hybrid The hybrid was prepared by mixing the prepared GO suspension and the yellow solution of HVO 3 at the desired ratio. The obtained dark yellow solution was aged in a glass container for 3 weeks to obtain a completely cured, homogeneous V 2 O 5 /GO hydrogel. The dried V 2 O 5 /GO xerogel was obtained by freeze drying the V 2 O 5 /GO hydrogel in a vacuum. The formed V 2 O 5 /GO xerogel was heated and annealed under N 2 at a rate of 5 °C min −1 up to 400 °C and kept constant at 400 °C for 6 h, during which the GO was reduced to graphene and the graphene-modified V 2 O 5 hybrid was formed. Electrochemical characterization The electrodes were prepared by casting a slurry of 80% V 2 O 5 –G, 10% polyvinylidence difluoride, and 10% carbon black onto a 10-μm-thick sheet of Al foil. For comparison, the pure V 2 O 5 ·nH 2 O was synthesized using the same conditions except for the addition of the GO. The corresponding electrodes were prepared using the same procedure. The prepared electrodes were placed in a vacuum oven and allowed to dry at 90 °C for 24 h. The electrolyte consisted of a solution of 1.2 M LiPF 6 (Novolyte, Ohio, USA) in a mixture of solvent from ethylene carbonate and ethyl methyl carbonate (EMC; 3:7, by weight; Novolyte, Ohio, USA). The prepared V 2 O 5 –G and V 2 O 5 were assembled into 2016-type coin cells using Li metal anodes (Aldrich, USA) and Celgard 3501 separators (Celgard, Ohio, USA) for characterizing their electrochemical performance. These cells were tested with an Arbin Battery cycler (BT-2000, Arbin, TX, USA) using different C-rates between 1.5 and 3.6 V. A Solartron 1287A/1260A Potentiostat/Impedance System (Solartron Analytical, England, UK) was used to measure the AC impedance of these cells in the frequency range of 0.01 Hz–1 MHz with an amplitude of 5 mV. The results were fitted using the model [28] , where R 0 is the contact resistance, R e and C e refer to the resistance and capacitance of the V 2 O 5 electrode, R ct and C dl stand for the charge-transfer resistance of the redox reaction of vanadium in V 2 O 5 and the double-layer capacitance in the electrode, respectively, and W d refers to the Warburg diffusion impedance, which could reflect the diffusion of Li ions in the V 2 O 5 . Materials characterization Scanning electron microscopy and energy-dispersive X-ray spectroscopy characterization were performed with a JEOL 7800 (Japan) operated at 5 kV. Standard high-resolution TEM characterization was performed with a JEOL 2100F (Japan) operated at 200 kV. Low-voltage (80 kV), aberration-corrected high-resolution TEM and EELS were conducted using a Titan 80/300 TEM. Cryogenic temperature TEM analysis was carried out for the synthesized V 2 O 5 hydrogel solutions with and without GO aged at different times to elucidate the formation mechanism. For the cryo-TEM, a 3.5-μl aliquot of the aged solution samples was placed on a copper grid (400 mesh) coated with a perforated/porous carbon film. The excess solution was blotted off with filter paper. The grid was then immediately plunged into liquid ethane cooled by liquid N 2 . After that, the sample grid was loaded into the microscope with a Gatan side-entry cryogenic holder. Low-dose images were collected using a CM 200 and CM 300 cryomicroscope with a field emission gun operating at 200 and 300 kV, respectively. The TGA was performed for both pure V 2 O 5 and V 2 O 5 –G using a TA 2000 thermoanalyzer. Temperature-dependent in operando HEXRD measurements during the annealing processes were performed on the beam line 11-ID-C at Advanced Photon Source, Argonne National Laboratory. A monochromator with a Si (311) single crystal was used to provide an X-ray beam with 115 keV of energy. A high-energy X-ray with a beam size of 0.2 × 0.2 mm and wavelength of 0.108 Å was used to obtain 2D diffraction patterns in the transmission geometry. X-rays were collected with a Perkin-Elmer large-area detector placed at 1,800 mm from the sample. The synthesized pure V 2 O 5 and V 2 O 5 –G were dried at 80 °C overnight and were pressed into pellets about 1-mm thick. The pellet was placed between a ceramic can and a platinum cover with a hole (D=1 mm) in the centre of both the can and the cover. After that, the ceramic can was placed vertically in a programmable furnace with glass windows, and nitrogen was used as the protective gas. The sample was heated up to 600 °C with a heating rate of 2 °C per minute. The diffraction data from the sample was collected every 34 s. The obtained 2D diffraction patterns were calibrated using a standard CeO 2 sample and converted to one-dimensional patterns using Fit2D software [62] . Synchrotron radiation-based in operando X-ray absorption spectroscopy can be very informative when applied to complex battery systems [63] . Particularly, the in operando XANES technique is very powerful for determining the average oxidation state and local structure of the elements in all phases. With these considerations in mind, we carried out in operando XANES measurements during the cycling of coin cells that contained the V 2 O 5 –G electrode on the beam line 20-BM-B at Advanced Photon Source, Argonne National Laboratory. Before the in operando synchrotron experiment, the XANES spectrum of the reference (commercial V 2 O 5 powder) was taken for comparison. As can be seen in Supplementary Fig. 5 , the XANES spectrum comparison between the commercial V 2 O 5 and the V 2 O 5 –G overlapped very well, suggesting that the intercalation did not cause a significant change in the valence state of the vanadium, which is consistent with the EELS results. The Li/V 2 O 5 coin cells with holes ( D =2 mm) at the centre were assembled for the in operando XANES study. The holes were sealed using Kapton tapes, which allowed the X-rays through but prevented air from entering the cell. In operando XANES was performed at the vanadium K-edge to monitor the change of the valence state of the vanadium in the cathode material. The XANES measurements were carried out in transmission mode at the beamline 20-BM-B of the APS using a Si (111) monochromator. Energy calibration was performed by using the first derivative point of the XANES spectrum for the V (K-edge=5463.76 eV). In the meantime, the reference spectra were collected for each in operando spectrum where vanadium metal was used in the reference channel. The coin cells with the exact same electrodes were also used because of the better signal-to-noise ratio. All cells were charged/discharged with a constant current of about 0.5 C between 1.7 and 3.6 V, while the XANES spectra data were collected every 262 s. The XANES data reduction and analysis followed standard methods using the ATHENA software package. How to cite this article : Liu, Q. et al . Graphene-modified nanostructured vanadium pentoxide hybrids with extraordinary electrochemical performance for Li-ion batteries. Nat. Commun. 6:6127 doi: 10.1038/ncomms7127 (2015).